The femur ofOrrorin tugenensisexhibits morphometric affinities with both Miocene apes and later hominins Orrorin tugenensis (Kenya, ca . 6 Ma) is one of the earliest putative hominins. Its proximal femur, BAR 1002′00, was originally described as being very human-like, although later multivariate analyses showed an australopith pattern. However, some of its traits (for example, laterally protruding greater trochanter, medially oriented lesser trochanter and presence of third trochanter) are also present in earlier Miocene apes. Here, we use geometric morphometrics to reassess the morphological affinities of BAR 1002′00 within a large sample of anthropoids (including fossil apes and hominins) and reconstruct hominoid proximal femur evolution using squared-change parsimony. Our results indicate that both hominin and modern great ape femora evolved in different directions from a primitive morphology represented by some fossil apes. Orrorin appears intermediate between Miocene apes and australopiths in shape space. This evidence is consistent with femoral shape similarities in extant great apes being derived and homoplastic and has profound implications for understanding the origins of human bipedalism. At least three putative hominins are recorded in the African late Miocene: Sahelanthropus tchadensis from Toros-Menalla (Chad, ca . 7 Ma) [1] ; Orrorin tugenensis from the Lukeino Formation (Kenya, ca . 6 Ma) [2] ; and Ardipithecus kadabba from the Middle Awash area (Ethiopia, ca . 5.5 Ma) [3] , the latter being followed closely in time by the early Pliocene Ardipithecus ramidus (4.4 Ma), for which a very complete skeleton is available [4] . The geographical and chronological distribution of these taxa strongly suggests that the earliest hominins evolved from an African Miocene ape. One of the earliest hallmarks of the human lineage is the adoption of habitual terrestrial bipedalism, which has been inferred for these fossil taxa on the basis of the foramen magnum position in Sahelanthropus [1] , proximal femoral anatomy in Orrorin [2] , [5] , [6] , [7] and pelvic and foot morphology in Ardipithecus [8] , [9] . The case of Orrorin is intriguing because its femur was originally described as being more modern human-like than that of later Plio-Pleistocene australopiths. This was interpreted—together with dental morphology—as evidence for a direct phylogenetic link between Orrorin and Homo to the exclusion of australopiths [2] , [5] (but see refs 10 , 11 for a different interpretation). Using multivariate statistics, Richmond and Jungers [6] concluded that BAR 1002′00 more closely resembled later australopiths in having a small head, a long and anteroposteriorly compressed neck and a wide proximal shaft; this suggested that these extinct taxa shared similar hip biomechanics that evolved early in hominin evolution. Among the three partial femora attributed to Orrorin —BAR 1002′00, 1003′00 and 1215′00 (refs 2 , 5 )—virtually all previous interpretations have been based on BAR 1002′00, which is the most complete specimen [2] , [5] , [6] , [7] , [12] . This femur, attributed to a young adult individual, preserves most of the proximal region and the shaft, although part of the greater trochanter is broken away slightly above its root. It has been previously noted that, because chimpanzees are humans’ closest relatives based on molecular data [13] , extant great apes are all too often the only non-human primates incorporated into hominin comparative analyses [14] . Thus, the commonality among most past studies of the BAR 1002′00 femur is that they employed qualitative and/or quantitative analyses to assess its morphological affinities with other fossil hominins within a comparative framework limited to extant great apes and humans. However, assuming a Pan -like ancestral morphotype for the hominin lineage may strongly misguide hypotheses on the actual pathway of human evolution. There is a growing body of evidence that not only humans but also extant great apes are highly derived taxa, having undergone millions of years of evolutionary change along divergent paths [11] , [14] , [15] , [16] ; in the case of chimpanzees, this has also been shown recently to be true at the genetic level [17] . Thus, it is possible that none of the extant taxa closely resemble the last common ancestor of living apes and humans. Taking into account that O. tugenensis is dated to the late Miocene, a broader comparative sample—including earlier Miocene apes—is necessary, as previously suggested [14] , to clarify and reliably interpret the morphology from which the earliest bipeds evolved. Extant apes constitute a relict of a once highly diversified group [18] , which in the Miocene was widely distributed throughout Africa and Eurasia. Relatively well-preserved skeletons are available for stem hominoids—interpreted as stem catarrhines by Harrison [11] —from the early ( Morotopithecus and Proconsul ) and middle ( Equatorius and Nacholapithecus ) Miocene of Africa [19] , [20] , [21] , [22] , as well as fossil great apes from the middle ( Pierolapithecus ) and late ( Hispanopithecus and Oreopithecus ) Miocene of Europe [23] , [24] , [25] . Pickford et al. [5] offered some qualitative comparisons of the Orrorin femora to Miocene apes but largely emphasized differences between the two groups (for example, neck length, gluteal tuberosity morphology and femoral anteversion). However, there are numerous and equally obvious similarities between Miocene apes and Orrorin , including the shape, size and orientation of the lesser trochanter, the laterally protruding base of the greater trochanter, the broad proximal shaft region, the size and shape of the head, as well as a laterally protruding gluteal tuberosity or small third trochanter. The latter feature has also been observed in the fragmentary proximal femur of Ar. ramidus and the Australopithecus afarensis femoral specimen from Maka [8] . Since this feature is present in some hylobatids, in some platyrrhines and even in Aegyptopithecus [26] , little doubt should remain about its primitiveness. Thus, an alternative—and as yet untested—morphological interpretation of the BAR 1002′00 femur is that it is not only temporally but also morphologically intermediate between Miocene apes and other early hominins. To assess the morphometric affinities of BAR 1002′00 with Miocene apes and fossil hominins among a large sample of extant anthropoids, we relied on three-dimensional geometric morphometric analyses (3DGM) of thirteen landmarks drawn from relevant regions preserved in BAR 1002′00, as well as some linear metrics derived from them. Similar approaches have been used to link particular morphological characteristics of the hominoid proximal femur with their observed locomotor patterns [27] and to evaluate the taxonomic affinities of early Plio-Pleistocene hominins [28] , [29] . This study differs in that it evaluates explicitly the morphological affinities of BAR 1002′00 within a broader comparative context that includes hylobatids, all extant great ape species, modern humans, early Plio-Pleistocene hominins, as well as four of the most complete Miocene ape proximal femora. Extant and fossil ape proximal femoral shape variation—and its covariation with size—was also explored within a large taxonomic sample of platyrrhine and cercopithecoid monkeys. We further inspected the phylogenetic structure of our morphometric data and modelled hominoid proximal femoral shape evolution by means of squared-change parsimony reconstruction of ancestral morphologies [30] . Finally, we examined two functionally relevant measures of the proximal femur: relative size of head and neck [31] and biomechanical neck length [32] , [33] . This study reveals that the femora of hominins and that of modern great apes evolved in different directions from a more primitive (that is, plesiomorphic) morphology that can be approximated by that of some Miocene apes. Our reconstruction of proximal femur shape evolution implies that the similarities shared by extant great ape genera are homoplastic and most probably related to suspensory behaviours. The femoral shape of Orrorin emerges as a unique mosaic that combines both Miocene ape and early hominin features, consistent with its age and the view that it was an incipient biped. Our results stress the need to incorporate fossil apes into analyses and discussions dealing with postcranial evolution in early hominins, especially those concerned with the emergence of human bipedalism. Principal patterns of variation among extant anthropoids The proximal femora of fossil apes, selected fossil hominins and extant hominoids are displayed in anterior ( Fig. 1 ) and lateral ( Supplementary Fig. S1 ) views, respectively. To assess and contextualize the shape affinities of the fossils within a large sample of extant anthropoid primates ( Supplementary Tables S1 and S2 ), we focused on thirteen 3D surface landmarks that capture much of overall proximal femoral shape ( Supplementary Fig. S2 ). Our principal components analysis with eigenanalysis computed on the extant anthropoid generic means (that is, between-group PCA; Fig. 2 ) reveals that when the two first components are inspected together (35% and 28.7% of the total variance, respectively), major taxonomic groups (that is, platyrrhines, cercopithecoids and hominoids) can be pulled apart. This fact suggests the presence of phylogenetic structure in our morphometric data (that is, more closely related taxa are also phenotypically more similar to each other than to more phylogenetically distant taxa). This is confirmed by a permutation test simulating the absolute absence of phylogenetic signal [34] in our anthropoid taxa tips (100,000 permutations, P <0.0001; Supplementary Fig. S3a ). When PC scores are computed a posteriori for all fossil specimens and plotted on the shape space previously defined by the extant anthropoids, fossils (Miocene apes, hominins and Orrorin ) occupy a similar position within hylobatids and/or humans. Although the statistical power to detect phylogenetic signal in the data diminishes with the reduced number of terminal taxa analysed [35] , it is still detected when examined among catarrhines only (100,000 permutations, P <0.001; Supplementary Fig. S3b ); or even when only the six cercopithecoid genera are analysed (100,000 permutations, P <0.05); Supplementary Fig. S3c ). However, phylogenetic structure is not detected when limited to the six extant hominoid genera ( Supplementary Fig. S3d ). 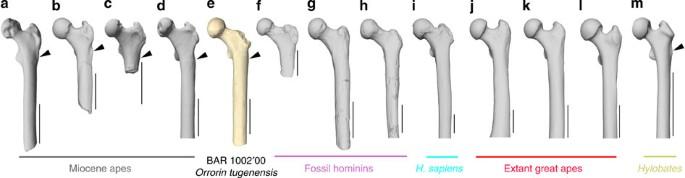Figure 1: Morphological comparison of BAR 1002′00 with selected proximal femora analysed in this study. (a) IPS 18800 (reversed),Hispanopithecus laietanus; (b) IPS 41724 (reversed), cf.Dryopithecus fontani; (c) BMNH-M-16331,Equatorius africanus; (d) KNM-MW 13142 A (reversed),Proconsul nyanzae; (e) BAR 1002′00,Orrorin tugenensis; (f) SK 97 (reversed),Paranthropus robustus; (g) A.L. 288-1,Australopithecus afarensis; (h) KNM-ER 1481, earlyHomo; (i)Homo sapiens; (j)Gorilla gorilla; (k)Pan troglodytes; (l)Pongo pygmaeus; and (m)Hylobates. The late Miocene specimen BAR 1002′00 (e) shares some features with later fossil hominins (f–h), such as a long and anteroposteriorly compressed neck and a spherical and small head. However, the femoral head morphology, the neck-shaft angle, the laterally flaring base of the greater trochanter and the medially expanded lesser trochanter resemble the morphology displayed by Miocene apes (a–d). The arrows indicate a laterally protruding gluteal tuberosity, observed inHylobates, Miocene hominoids, as well as inOrrorinandArdipithecus ramidus8. All specimens are scaled to similar mediolateral breadth. Scale bars represent 5 cm. Figure 1: Morphological comparison of BAR 1002′00 with selected proximal femora analysed in this study. ( a ) IPS 18800 (reversed), Hispanopithecus laietanus ; ( b ) IPS 41724 (reversed), cf. Dryopithecus fontani ; ( c ) BMNH-M-16331, Equatorius africanus ; ( d ) KNM-MW 13142 A (reversed), Proconsul nyanzae ; ( e ) BAR 1002′00, Orrorin tugenensis ; ( f ) SK 97 (reversed), Paranthropus robustus ; ( g ) A.L. 288-1, Australopithecus afarensis ; ( h ) KNM-ER 1481, early Homo ; ( i ) Homo sapiens ; ( j ) Gorilla gorilla ; ( k ) Pan troglodytes ; ( l ) Pongo pygmaeus ; and ( m ) Hylobates . The late Miocene specimen BAR 1002′00 ( e ) shares some features with later fossil hominins ( f – h ), such as a long and anteroposteriorly compressed neck and a spherical and small head. However, the femoral head morphology, the neck-shaft angle, the laterally flaring base of the greater trochanter and the medially expanded lesser trochanter resemble the morphology displayed by Miocene apes ( a – d ). The arrows indicate a laterally protruding gluteal tuberosity, observed in Hylobates , Miocene hominoids, as well as in Orrorin and Ardipithecus ramidus [8] . All specimens are scaled to similar mediolateral breadth. Scale bars represent 5 cm. 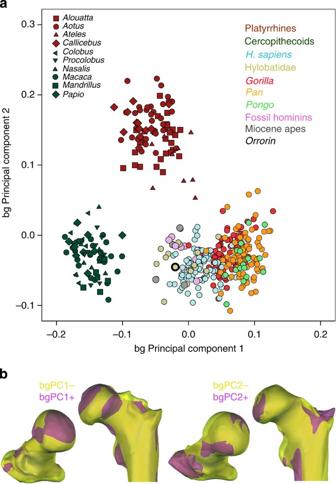Figure 2: Principal patterns of proximal femur shape variation amongst extant anthropoids. (a) The bivariate plot of the two first axes of the between-group principal components analysis (bgPCA, representing 35% and 28.7% of the total variance respectively) indicates that platyrrhine, cercopitecoid and hominoid extant proximal femora can be characterized. When fossil ape and hominin femora are situated in the shape space defined by the extant taxa, they all fall within the extant hominoid cloud, especially nearH. sapiensand hylobatids. (b) Warped surfaces (based on a thin-plate spline) were superimposed for each axis: bgPC1 represents values of −0.10 (yellow) and +0.10 (purple); bgPC2 representes values of −0.05 (yellow) and +0.10 (purple). Full size image Figure 2: Principal patterns of proximal femur shape variation amongst extant anthropoids. ( a ) The bivariate plot of the two first axes of the between-group principal components analysis (bgPCA, representing 35% and 28.7% of the total variance respectively) indicates that platyrrhine, cercopitecoid and hominoid extant proximal femora can be characterized. When fossil ape and hominin femora are situated in the shape space defined by the extant taxa, they all fall within the extant hominoid cloud, especially near H. sapiens and hylobatids. ( b ) Warped surfaces (based on a thin-plate spline) were superimposed for each axis: bgPC1 represents values of −0.10 (yellow) and +0.10 (purple); bgPC2 representes values of −0.05 (yellow) and +0.10 (purple). Full size image Shape differences in bgPC1 are correlated with larger heads relative to neck height in hominoids, which also exhibit more spherical heads in comparison with cercopithecoid monkeys. The latter have a proximodistally high neck and a head in which the proximolateral-to-distomedial diameter predominates over its orthogonal dimension. Cercopithecoid femora also exhibit anterior portions of the greater trochanter base extending more medially and anteriorly. The positive values of this axis are occupied by the extant great apes, while modern humans, and especially hylobatids, occupy an intermediate position along the axis, largely overlapping with the platyrrhine monkey range and especially with Ateles. Positive values of this axis are also correlated with slightly smaller lesser trochanters. bgPC2 largely separates platyrrhine from catarrhine anthropoids. Again, the exceptions are two Ateles individuals overlapping with two Pan specimens. The positive values along this axis displayed by platyrrhine anthropoids are correlated with slightly smaller (less anterolaterally extending) heads, differences in greater trochanter morphology, in which the most lateral point is more proximally situated and the most anterior point extends more medially, as well as in lesser trochanter, extending slightly less medially and proximally. Regression of shape on log-transformed centroid size (CS; representing proximal femur size) shows a significant correlation (10,000 permutations, P <0.05), although only accounts for 7.1% of total shape variation. This relationship becomes non-significant when phylogenetic independent contrasts (PICS) are used instead of terminal taxa (TIPS). This indicates that major shape differences in the proximal femora between extant anthropoids cannot be ‘explained’ by differences in femoral size. Principal patterns of variation among extant hominoids After discovering that fossil hominoids show their closest shape affinities within modern apes and humans, we repeated the previous analysis focusing only on modern hominoids to maximize and visualize their femoral shape variation. Scores for extant individuals and fossil specimens were computed post hoc and plotted in the extant hominoid shape space ( Fig. 3 ). bgPC1 (46.1% of variance) is correlated with the base of the greater trochanter shape and orientation, shape of the head, its position relative to the lesser trochanter and the distal extension of the latter. Thus, great apes and especially Pan (the latter with the most negative values on this axis) show a proximally oriented base of the greater trochanter (both most anterior and most lateral points), with a concomitantly deeper fossa trochanterica, and a head with a predominantly anteroposterior dimension oriented more anteriorly relative to the lesser trochanter. By contrast, positive values of bgPC1 in modern humans and hylobatids (together with some gorilla specimens) are correlated with a greater trochanter base that extends more laterally as well as more anteriorly on the medial side of the base, thus being lower relative to the head. Furthermore, the lesser trochanter extends slightly more distally and is more anteriorly oriented relative to the head. Most Gorilla and Pongo specimens occupy an intermediate position on this axis. 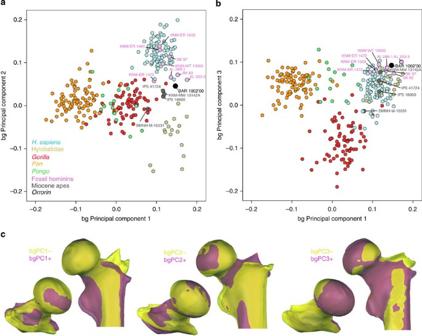Figure 3: Principal patterns of proximal femur shape variation among extant hominoids. This between-group principal components analysis (bgPCA) iterated in modern hominoids only shows that when the first principal axes of shape variation are considered together, overall, extant great ape genera and modern humans can be distinguished by the morphology of their proximal femur. (a) bgPC1 (46.1% of variance) and bgPC2 (27% of variance); (b) bgPC1 and bgPC3 (19.4% of variance). When fossil ape and hominin femora are situated in the shape space defined by the extant taxa, most Miocene fossils occupy a similar position to each other, which is similar to that ofOrrorinand other hominins. (c) Warped surfaces (based on a thin-plate spline) were superimposed for each axis: bgPC1 and bgPC2 represent values of −0.10 (yellow) and +0.10 (purple); bgPC3 represents values of −0.10 (yellow) and +0.05 (purple). Figure 3: Principal patterns of proximal femur shape variation among extant hominoids. This between-group principal components analysis (bgPCA) iterated in modern hominoids only shows that when the first principal axes of shape variation are considered together, overall, extant great ape genera and modern humans can be distinguished by the morphology of their proximal femur. ( a ) bgPC1 (46.1% of variance) and bgPC2 (27% of variance); ( b ) bgPC1 and bgPC3 (19.4% of variance). When fossil ape and hominin femora are situated in the shape space defined by the extant taxa, most Miocene fossils occupy a similar position to each other, which is similar to that of Orrorin and other hominins. ( c ) Warped surfaces (based on a thin-plate spline) were superimposed for each axis: bgPC1 and bgPC2 represent values of −0.10 (yellow) and +0.10 (purple); bgPC3 represents values of −0.10 (yellow) and +0.05 (purple). Full size image bgPC2 (27% of variance; Fig. 3a ) is correlated with greater trochanter basal shape and orientation, head shape and orientation and lesser trochanter proximomedial expansion. Negative values of bgPC2 are correlated with a greater trochanter with a base whose more anteromedial and most lateral points are close in the vertical dimension, both anteriorly oriented and the lateral point also more laterally protruding. Negative values are also correlated with a proximomedially expanded (that is, larger) lesser trochanter (larger intertrochanteric diameter). Conversely, positive values of bgPC2 are correlated with a proximolateral orientation of the greater trochanter base, whose most lateral point is situated more inferiorly relative to the head, a smaller lesser trochanter and a head that is slightly more medially oriented. All extant great apes occupy an intermediate position on this axis, whereas most humans have high values on the axis and overlap with few apes (four Pan , one Pongo and two Gorilla specimens). Some hylobatids have negative values on this axis. When the shape space defined by bgPC1 and bgPC2 is inspected ( Fig. 3a ), modern humans and hylobatids do not overlap with the remaining extant apes, and fossil hominins are within or immediately around the human cloud. The proximal femora of Proconsul, Dryopithecus and Hispanopithecus occupy virtually the same position in bgPC1 similar to hylobatids, modern humans and fossil hominins, respectively. These three Miocene specimens are also very close in bgPC2, overlapping with all great apes. The Equatorius femur is slightly different from other Miocene specimens with slightly lower values of both bgPC1 and bgPC2, being on the margin but within the Gorilla cloud. Orrorin is situated on the upper margin of the modern human range for bgPC1 and close to the upper margin of the extant great ape range for bgPC2 being intermediate between fossil hominins and three of the Miocene ape specimens. Negative values of bgPC3 (19.4% of variance; Fig. 3b ) separate most Gorilla individuals by virtue of the higher position of their greater trochanter base relative to the head (which could be related to their lower collodiaphyseal angle [36] ). Furthermore, the gorilla femoral head extends less proximomedially in relation to their more hemispherical head shape. When Procrustes distances between centroid fossils and extant taxa are compared ( Supplementary Table S4 ), the femur of Orrorin (BAR 1002′00) exhibits its closest shape affinities to that of Proconsul nyanzae (KNM-MW 13142 A) and secondarily to both femora of Au. afarensis (AL 333-3 and AL 288-1). Regression of hominoid proximal femoral shape on log CS (including fossils) shows a non-significant relationship (using either PICS or TIPS). Similarly, within anthropoids, this indicates that shape differences in hominoid proximal femora are not explained simply by differences in femoral size, which is obvious when comparing modern humans with hylobatids (that is, similar bgPC1 scores in spite of the large size differences). Phylomorphospace of hominoid proximal femur evolution To inspect the major changes in proximal femoral shape during hominoid evolution, we constructed a morphospace (shape space in this case) defined by the two first axes of a PCA of the covariance matrix of extant and extinct hominoid taxa means. A phylogenetic tree ( Fig. 4 ) was mapped onto it by reconstructing hypothetical ancestral morphologies (that is, internal nodes) using squared-change parsimony [30] . This PCA slightly differs from the previous one in that fossil species do participate in the characterization of the shape space, and thus shape variation among fossil hominoids is now comparable to that displayed by extant great apes ( Fig. 5 ). PC1 (37.5% of variance) is correlated with the following: position, width and orientation of the greater trochanter base; relative size, shape and orientation of the head; anatomical neck length; and lesser trochanter size and orientation. PC2 (17.8% of variance) is correlated also with size and orientation of the lesser trochanter, the shape of the head, as well as the position of the anterior portion of the base of the greater trochanter and its most lateral extension. 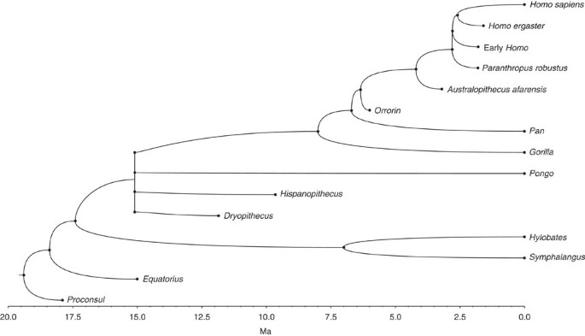Figure 4: Phylogenetic tree of the extant and fossil hominoids analysed in this study. The tree is based on molecular data available for extant taxa incorporating fossil specimens by using information from different sources. Figure 4: Phylogenetic tree of the extant and fossil hominoids analysed in this study. The tree is based on molecular data available for extant taxa incorporating fossil specimens by using information from different sources. 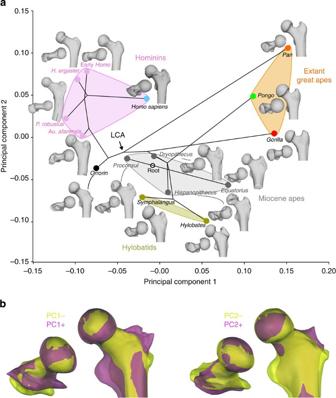Figure 5: Phylomorphospace of hominoid proximal femur evolution. (a) The phylogeny presented inFigure 4is projected into a plot defined by the two first principal components (PC's) of the covariance matrix among extant genera and fossil species means (PC1=32.9% and PC2=18.5% of the total variance, respectively). Internal node morphologies were reconstructed using squared-change parsimony, and branch lengths were derived from estimated divergence times. (b) Warped surfaces (based on a thin-plate spline) representing shape changes associated with each axis were superimposed: PC1 represents values of −0.15 (yellow) and +0.15 (purple); PC2 represents values of −0.10 (yellow) and +0.10 (purple). To facilitate the morphospace interpretation, 3D surfaces representing extant and fossil species were plotted (Au. afarensisis represented by AL 288-1 ‘Lucy’;P. robustusis represented by SK 82, reversed; earlyHomois represented by KNM-ER 1481). Hand-drawn ellipses indicate major shape groups. Phylogenetic structure is not found in the phylomorphospace of hominoid proximal femora, as indicated by our permutation test against the null hypothesis of complete lack of phylogenetic signal (100,000 permutations,P=0.148). Full size image Figure 5: Phylomorphospace of hominoid proximal femur evolution. ( a ) The phylogeny presented in Figure 4 is projected into a plot defined by the two first principal components (PC's) of the covariance matrix among extant genera and fossil species means (PC1=32.9% and PC2=18.5% of the total variance, respectively). Internal node morphologies were reconstructed using squared-change parsimony, and branch lengths were derived from estimated divergence times. ( b ) Warped surfaces (based on a thin-plate spline) representing shape changes associated with each axis were superimposed: PC1 represents values of −0.15 (yellow) and +0.15 (purple); PC2 represents values of −0.10 (yellow) and +0.10 (purple). To facilitate the morphospace interpretation, 3D surfaces representing extant and fossil species were plotted ( Au. afarensis is represented by AL 288-1 ‘Lucy’; P. robustus is represented by SK 82, reversed; early Homo is represented by KNM-ER 1481). Hand-drawn ellipses indicate major shape groups. Phylogenetic structure is not found in the phylomorphospace of hominoid proximal femora, as indicated by our permutation test against the null hypothesis of complete lack of phylogenetic signal (100,000 permutations, P =0.148). Full size image Branch lengths indicate that similar evolutionary shape changes (as characterized by PC1) have occurred independently in the three extant great ape lineages ( Pongo, Gorilla and especially Pan ). Those morphological changes are largely characterized by narrowing and more proximal orientation of the greater trochanter base (being also higher relative to the head) and slight enlargement of head diameter relative to proximal femoral dimensions. The fossil ape Equatorius just approaches the extant great ape configuration on PC1. Conversely, early hominins—as evidenced by Orrorin , australopiths, early Homo and Homo ergaster —experienced less marked changes than extant great apes did in PC1 (as compared relative to the position of the hominoid root): their greater trochanter base has a more vertical orientation and is situated lower relative to the head (especially its more lateral point); they display a longer anatomical neck; their femoral heads are smaller, especially the junction with the neck, which could be related to the head articular surface covering a larger portion of a sphere; the head has also a more medial set on the neck; and, finally, their lesser trochanters are less conspicuous and situated more posteriorly relative to the head. Hylobatids are close to Miocene hominoids and modern humans in PC1. Less marked proximal femoral shape changes (as accounted by PC2) explain the evolution of the crown group of extant great apes, modern humans and fossil hominins. These morphological changes are more accentuated in Pan than in Pongo and modern humans (and only slightly noticeable in Gorilla ) and include the following: lesser and greater trochanter extend less medially and laterally, respectively (that is, narrower intertrochanteric length); changes in the relative position of the most anterior portion of the greater trochanter base (it is more proximally situated and less anteriorly protruding); and subtle changes in head shape (similarly as changes associated with PC2 in the previous analysis, reported in Fig. 3 ). Hylobatids depart slightly from the Miocene ape condition in the opposite direction from extant great apes and hominins (that is, negative values of PC2). Hispanopithecus is the fossil ape with closest affinities to hylobatids in this axis. When inspected together, both axes separate extant great apes from fossil apes, hylobatids and hominins. The Orrorin specimen is most similar to early hominins in PC1 and most similar to Miocene apes in PC2. Using squared-change parsimony, the reconstructed proximal femur of the last common ancestor of Pan and hominins (LCA) is close in shape space to Proconsul. As far as hominin proximal femoral evolution is concerned, from the inferred morphology of the LCA, Orrorin exhibits changes in PC1 towards the hominin direction (for example, anatomical neck length, low position of greater trochanter base relative to a slightly smaller head comprising a major portion of a sphere). Major morphological changes over time from Orrorin into australopiths ( Au. afarensis plus Paranthropus robustus ) and subsequently into early fossil Homo are traced by increased values on PC2 (for example, reduction in medial expansion of lesser trochanter, intertrochanteric distance, changes on greater trochanter base and head shape). Paranthropus robustus is extreme for negative values of PC1. From this Plio-Pleistocene hominin configuration, Homo sapiens has experienced small modifications on its proximal femur, as accounted by increased values of PC1 (that is, slightly larger heads, with less symmetrically covered articular surface, more proximally situated and medially extending base of greater trochanter, slightly larger lesser trochanter). Head size relative to neck height When head size (approximated by its CS) is compared with neck height ( Fig. 6 ; Supplementary Table S5 ), all modern hominoids show a clearly different pattern in which their heads are relatively larger than in any extant catarrhine or platyrrhine monkey genera analysed ( F- test, P <0.001). However, the upper ranges of Macaca and Alouatta overlap with the lower ranges of all extant hominoids, with the exception of Pongo. Although all monkey genera overlap in their ranges to some extent, Ateles and Alouatta display a clear tendency to have larger heads than the remaining anthropoid monkeys, with significant differences from Callicebus and Aotus ( P ≤0.001). Alouatta, with a larger sample than Ateles , further shows significantly larger heads than Papio ( F- test, P =0.005), Procolobus ( F- test, P =0.001) and Colobus ( F- test, P <0.001). The ranges of all extant hominoids do also largely overlap. However, Pongo clearly has the largest head relative to neck height ( F- test, P <0.001), although this might be partially caused by the lack of fovea capitis (that is, less invaginated landmark 1). The ranges of hylobatids, and to a lesser extent Pan , are slightly higher than in Gorilla and H. sapiens . The four fossil apes investigated are within the low range of modern hominoids, with the exception of Hispanopithecus , which is within the interquartile distribution of Pongo (and the upper range of the remaining hominoids, even having a deep fovea capitis ). Equatorius also falls within the uppermost range of Alouatta and Macaca . The majority of fossil hominins investigated fall within the modern human range, also overlapping with the non- Pongo hominoid distribution (by excluding its single outlier). KNM-ER 1503, SK 97 and SK 82 (in this order, the latter falling right below the extant ape and human distribution) show the smallest heads, overlapping also with the uppermost ranges of Alouatta and Macaca . 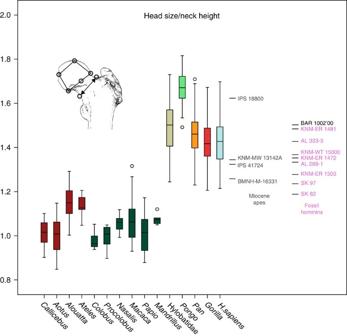Figure 6: Femoral head size relative to neck height. Overall, extant and extinct hominoids have larger heads relative to neck than extant platyrrhine and cercopithecoid monkeys. The inset drawing represents the landmarks employed to compute the femoral head CS and neck height. Boxplots represent 25th and 75th percentiles, respectively, centre line is the median, whiskers represent non-outlier range and dots are outliers. Samples for each boxplot areCallicebus(n=14), Aotus(n=15),Alouatta(n=30),Ateles(n=9),Colobus(n=9),Procolobus(n=8),Nasalis(n=8), Macaca(n=26),Papio(n=10),Mandrillus(n=6), Hylobatidae (n=16),Pongo(n=16),Pan(n=88),Gorilla(n=77),H. sapiens(n=87). Figure 6: Femoral head size relative to neck height. Overall, extant and extinct hominoids have larger heads relative to neck than extant platyrrhine and cercopithecoid monkeys. The inset drawing represents the landmarks employed to compute the femoral head CS and neck height. Boxplots represent 25th and 75th percentiles, respectively, centre line is the median, whiskers represent non-outlier range and dots are outliers. Samples for each boxplot are Callicebus ( n =14) , Aotus ( n =15), Alouatta ( n =30), Ateles ( n =9), Colobus ( n =9), Procolobus ( n =8), Nasalis ( n =8) , Macaca ( n =26), Papio ( n =10), Mandrillus ( n =6), Hylobatidae ( n =16), Pongo ( n =16), Pan ( n =88), Gorilla ( n =77), H. sapiens ( n =87). Full size image Biomechanical neck length When the biomechanical neck length (BNL) is measured relative to proximal femur size (approximated by the CS; Fig. 7 ; Supplementary Table S6 ), modern humans have longer BNL than extant great apes ( F- test, P <0.001) and hylobatids ( F- test, P <0.01). Although extant great apes and humans have clearly different interquartile distributions, there is an overlap between the upper ranges of the three extant great ape genera and the lower ranges of humans. Hylobatids show a more intermediate distribution between humans and great apes and are statistically different from chimpanzees ( F- test, P <0.01) and gorillas ( F- test, P =0.05) but not from Pongo ( F- test, P =1.0). However, when compared with our comparative sample of anthropoid monkeys, modern humans do not show significantly longer BNL than Mandrillus, Procolobus, Alouatta, Aotus and Callicebus . All fossil specimens (fossil hominins as well as the four Miocene apes) fall within the human range, with the notable exceptions of Orrorin and KNM-ER 1503, both being above the ranges of modern humans and other anthropoid taxa analysed. When excluding outliers, the four Miocene hominoids examined have BNLs above the extant great ape range. These results suggest that the short BNLs displayed by some extant catarrhine primates, and especially extant African apes, could be the exception (that is, the derived ones) instead of the rule. 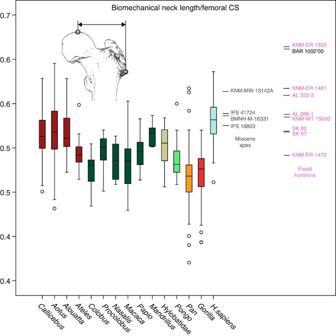Figure 7: Biomechanical neck length. Relative to proximal femoral centroid size, and in spite of a large overlap with some monkeys, modern humans have longer biomechanical necks than other anthropoid primates, and especiallyPan. All Miocene hominoids and fossil hominins fall within the modern human distribution, with the exception of BAR 1002′00 (Orrorin tugenensis) and KNM-ER 1503 (Paranthropus boisei/Homosp.). The inset drawing represents the biomechanical neck length of the femur. Boxplots represent 25th and 75th percentiles, respectively, centre line is the median, whiskers represent non-outlier range and dots are outliers. Samples for each boxplot areCallicebus(n=14),Aotus(n=15),Alouatta(n=30),Ateles(n=9),Colobus(n=9),Procolobus(n=8),Nasalis(n=8),Macaca(n=26),Papio(n=10),Mandrillus(n=6), Hylobatidae (n=16),Pongo(n=16),Pan(n=88),Gorilla(n=77),H. sapiens(n=87). Figure 7: Biomechanical neck length. Relative to proximal femoral centroid size, and in spite of a large overlap with some monkeys, modern humans have longer biomechanical necks than other anthropoid primates, and especially Pan . All Miocene hominoids and fossil hominins fall within the modern human distribution, with the exception of BAR 1002′00 ( Orrorin tugenensis ) and KNM-ER 1503 ( Paranthropus boisei / Homo sp.). The inset drawing represents the biomechanical neck length of the femur. Boxplots represent 25th and 75th percentiles, respectively, centre line is the median, whiskers represent non-outlier range and dots are outliers. Samples for each boxplot are Callicebus ( n =14), Aotus ( n =15), Alouatta ( n =30), Ateles ( n =9), Colobus ( n =9), Procolobus ( n =8), Nasalis ( n =8), Macaca ( n =26), Papio ( n =10), Mandrillus ( n =6), Hylobatidae ( n =16), Pongo ( n =16), Pan ( n =88), Gorilla ( n =77), H. sapiens ( n =87). Full size image Our results show that extant anthropoid taxonomic groups can be distinguished by means of the major patterns of shape variation of their proximal femora ( Fig. 2 ), thereby indicating the presence of phylogenetic structure in the morphometric data ( Supplementary Fig. S3a ). However, when comparing the same number of terminal taxa in extant cercopithecoids and hominoids independently, the former still exhibit a significant phylogenetic signal ( Supplementary Fig. S3c ), whereas hominoids fail to reveal phylogenetic structure ( Supplementary Fig. S3d )—with similar results when including fossil apes and hominins ( Fig. 5 ). Insights into adaptive radiations can be extracted by comparing the phylogenetic structure in morphometric data present in different subclades [35] . Thus, our results suggest that, in comparison with cercopithecoid monkeys, hominoids have a higher diversity of proximal femoral morphologies, and that similarities between extant great apes are homoplastic ( Fig. 5 ). Importantly, when principal component scores are computed for fossil apes on the basis of a shape space defined by extant anthropoids, they show their closest affinities with modern apes ( Fig. 2 ). Although with some overlap with atelines, extant and extinct hominoids are characterized by the possession of a large head relative to neck height (PC1 axis in Fig. 2 ). The latter fact is confirmed by a specific analysis of femoral head CS relative to neck height ( Fig. 6 ). A large femoral head relative to neck size has been hypothesized as being indicative of greater hip mobility by allowing larger joint excursion (more specifically abduction) [31] . If this is indeed the case, our results indicate an adaptive shift towards enhanced mobility at the hip joint in hominoids relative to non-hominoid anthropoids that was already present by the early Miocene (as evidenced by Proconsul ). These results expand previous analyses indicating significantly larger heads relative to neck in great apes as compared with Macaca [31] , as well as inferences derived from femoral morphology in Miocene hominoids [19] , [36] , [37] , [38] , [39] . Conversely, the primitive pelvis of Proconsul [19] suggests mosaic evolution across both sides of the hominoid hip joint. When inspecting proximal femoral shape variation in extant hominoids only ( posteriori plotting of fossils; that is, their variation is not explored), extant hominid genera and hylobatids can be further distinguished ( Fig. 3 ). Fossil hominins are most similar to each other and to modern humans, while Proconsul, Dryopithecus and Hispanopithecus occupy a similar position of the shape space, overlapping with hylobatids and hominins (modern and fossils) in bgPC1 and with extant great apes in bgPC2. Although Miocene apes show closer shape affinities to modern hominoids than to modern monkeys ( Fig. 2 ), when compared with hominoids only ( Fig. 3 ), similarities between Miocene hominoids in shape space also support the idea that these taxa are more similar to each other than to any modern taxa [40] . When ape and hominin proximal femoral evolution is reconstructed using squared-change parsimony weighting by branch lengths and calibrating with fossils and molecular data ( Fig. 4 ), it appears that hominins and extant great apes have evolved in opposite directions from a morphology similar to that displayed by some Miocene apes ( Fig. 5 ). The last common ancestor of chimpanzees and humans (LCA) is reconstructed as having a proximal femoral external morphology very similar to that of Proconsul . Although the proximal femur of Orrorin shows its closest shape affinities with Proconsul ( Supplementary Table S4 ), it foreshadows the early hominin condition by ca . 6 Ma (PC1 in Fig. 5 ), as evidenced by its longer anatomical neck and its lower position of the greater trochanter base relative to its small head comprising a more complete sphere. Strikingly, Orrorin, Miocene hominoids and Hylobates show a modern human-like lateral protrusion of the greater trochanter, suggesting that Plio-Pleistocene hominins (specially australopiths) and extant great apes are (opposite) outliers in this respect. The biomechanical neck length (BNL) determines the moment arm of the lesser gluteals during the pelvic support phase of bipedal gait [32] , [33] . Thus, a long BNL could be potentially used as a highly diagnostic human feature since it would imply a reorientation of the line of action of these anterior muscles compared with apes. Although the BNL of the femoral neck should be measured relative to femoral length to evaluate its relevance during bipedalism [32] , [33] , and interpreted within the ‘total morphological pattern’ [33] , it is still relevant (and more feasible with available fossils) to compare its dimensions across a large comparative sample relative to proximal femoral size ( Fig. 7 ). Although overlap exists, humans do actually have a distinctive pattern relative to extant great apes. Fossil hominins and Miocene hominoids inspected all fall within the human range (with the exception of Orrorin and KNM-ER 1503, which fall slightly above), as well as some catarrhine and platyrrhine monkeys. This suggests that long BNL could be plesiomorphic for anthropoids, having been subsequently co-opted for enhanced lateral balance during bipedal locomotion in hominins. In contrast, extant great apes display proximally oriented greater trochanters ( Figs 3 and 5 ), which would enable the femur to move in a wider range of positions, in particular including the abducted postures that are more suitable for climbing, suspensory and other arboreal behaviours [33] , [41] , [42] . This great ape-like morphology of the greater trochanter, together with their high neck-shaft angle (characteristic of modern hominoids), could be in part responsible for their secondarily shortened BNL [32] . Chimpanzees show the most disparate morphology in shape space in comparison with hominins ( Figs 3 and 5 ), corroborating a previous analysis [28] and suggesting that the proximal femoral shape of Pan is very derived from the ancestral hominoid condition. This fact, which is reinforced by our evolutionary reconstruction since the LCA ( Fig. 5 ), might be related to the more derived (that is, cranially expanded) lower ilium of chimpanzees [8] . Although the nature of our morphometric approaches differs from previous analyses (for example, 3D coordinates instead of linear measurements [6] , [32] , [33] , [42] , different coordinate configuration [27] , [28] , [29] , no inclusion of proximal shaft dimensions [6] , [29] , [42] ), our results match and reinforce many of the conclusions from most previous analyses [6] , [28] , [43] , [44] , [45] by showing subtle differences between australopiths and fossil Homo (our PC2 in Fig. 5 ) in terms of proximal femoral shape. Our results also agree that Orrorin shows an external femoral anatomy more similar to that of early hominins than to that of modern humans [6] (PC1 in Fig. 5 ). However, by virtue of adding earlier Miocene apes, our results expand previous conclusions reached on Orrorin [2] , [5] , [6] by indicating that the six-million-year-old BAR 1002′00 femur is not modern human-like or intermediate between extant great apes and humans, but rather intermediate between more plesiomorphic fossil apes (as indicated by PC2 in Fig. 5 ) and Plio-Pleistocene hominins (as indicated by PC1 in Fig. 5 ). Our ancestral state reconstruction reveals that some Miocene apes might represent a more appropriate model for the ancestral morphology (at least for the proximal femur) from which hominins evolved than do extant great apes and especially the highly derived Pan (see also ref. 16 ). The modern human proximal femur, being adapted for obligate terrestrial bipedalism, differs slightly from that of early hominins (for example, larger head, shorter anatomical neck and less posteriorly oriented lesser trochanter; Fig. 5 ). Moreover, it has a greater trochanter that protrudes laterally beyond its base ( Fig. 1i ). This feature that has been explained as a medial shift of the relative position of the femoral shaft (relative to australopiths) to reduce the length of the anatomical neck (and thus its bending moment) while preserving a long biomechanical neck length (and thus not compromising the lever arm of the abductors for lateral balance) [32] . The modern human morphology, with its larger head, has been functionally linked to the need for withstanding a greater proportion of vertically transmitted body weight during bipedalism as compared with other types of locomotion [31] , [46] . The low and laterally projecting greater trochanter, in turn, helps to put the lesser gluteal muscles ( gluteus minimus and gluteus medius ) in the mechanically most advantageous positions during the stance phase: it translates the line of action of the horizontal component of the abductors to a more inferior position relative to head and neck, reducing the bending moment during abductory contractions. In addition, its lateral position increases the biomechanical neck length, while still allowing for considerable mobility at the hip joint [32] , [33] , [41] , [42] , [47] . Differences in femoral morphology between australopiths and humans have been interpreted by most authors as reflecting nontrivial differences in biomechanics at the hip joint during bipedalism [6] , [28] , [42] , [44] . Alternatively, other authors have argued that the hip biomechanics of australopiths and humans are essentially the same, so that the above-mentioned femoral differences are linked instead to correlated differences in pelvic geometry resulting from encephalization and details of child birth in Homo (also referred to as the ‘obstetrical dilemma’) [33] , [48] . In terms of origins of human bipedalism, apart from the morphometric resemblances of the external morphology of BAR 1002′00 with hominins found here and other studies [5] , [6] , [7] (for example, long and anteroposterioly flat anatomical neck, long biomechanical neck, small and spherical head, low position of greater trochanter relative to head), the Orrorin femur is also characterized by a proto- linea aspera , an obturator externus groove and a distribution of cortical bone in the femoral neck, which collectively are consistent with enhanced facultative bipedalism (as compared with fossil and modern apes) as early as 6 Ma [2] , [5] , [6] , [7] , [14] . However, the internal structure of BAR 1002′00 remains controversial in part due to the low resolution of the published CT-scan images [49] . A more recent re-analysis of the original BAR 1002′00 CT data, based on a limited comparative sample of chimpanzees and humans, led to conclude that the skewness of femoral cortical bone distribution at the midneck in BAR 1002′00 is more similar to that of chimpanzees than to that of humans, although less so when approaching the neck-shaft junction [12] . Interestingly, a recent study comparing the cortical neck distribution at the midneck and closer to the shaft has found a similar pattern in South African australopith femora [50] . Overall, differences in internal and external morphology in Orrorin specifically and australopiths in general relative to modern humans provide evidence of an altered gait due to the lack of a fully-developed, modern human-like abductor apparatus [6] , [12] , [50] . A different mode of bipedalism (from that of modern humans) practised by Orrorin (and Ar. ramidus ) is consistent with the possession of a laterally protruding gluteal tuberosity below the greater trochanter (that is, small third trochanter, for insertion of the ascending tendon of the gluteus maximus [51] ) in combination with a ‘broad proto- linea aspera ’ [5] , [8] . The latter arrangement indicates that a modern human configuration, consisting in a more posteromedial translation of the gluteus maximus insertion (functionally related to hypertrophy of the quadriceps at the expense of the hamstrings), had not yet occurred in the above-mentioned taxa [8] . Overall, our results agree with Napier’s [45] viewpoint, according to which the morphological pattern of the proximal femur displayed by some Miocene apes is more likely to have been co-opted for bipedalism than the derived femoral morphology that is displayed by extant great apes. This does not necessarily imply a particularly close phylogenetic link between hominins and some of the Miocene apes included in our analyses. Rather, it would imply that Miocene apes would closely resemble the femoral morphotype of the last common ancestor between African apes and hominins ( Fig. 5 ), whereas the morphology displayed by extant great apes would be much more derived—and probably homoplastic—as an adaptation for enhanced abduction during suspensory behaviours [8] , [16] , [41] . Similarly, parallel evolution has also been used to explain the similar, but not identical, trunk and forelimb morphologies within extant hominoids [52] . All Miocene apes considered within this study, including the more suspensory Hispanopithecus [24] that shows some hylobatid affinities in its femur ( Fig. 5 ), have been interpreted as displaying a significant arboreal quadrupedal component in their locomotor repertoires, although probably differing from that of extant monkeys [19] , [38] , [39] , [53] . Rose stated: ‘the fact of the ubiquity of quadrupedalism as a major locomotor mode in Miocene catarrhines in general, and Miocene hominoids in particular, is an inevitable starting point for any attempt to reach a full understanding of the emergence of the suspensory, quadrumanous climbing, quadrupedal-climbing-suspensory and bipedal specializations of extant hominoids’ [54] . This agrees with claims that the mechanical requirements imposed by quadrupedalism and bipedalism are more similar to each other than to those related to suspension [37] , [55] . Our results therefore support a modified version of the evolutionary scenario that early bipeds might have evolved from a more generalized arboreal, largely orthograde (but not specifically suspensory) Miocene ape [11] , [14] , [15] , [25] , [45] , with a more plesiomorphic postcranium than that exhibited by any of the extant African apes [8] , [16] . Femora samples used in the study Our total extant sample ( N =422) includes all the species of extant great apes and a selection of hylobatids ( Supplementary Table S2 ). Landmark data were collected on adult specimens (wild-shot extant non-human taxa) with full epiphyseal closure. Data were collected on original fossils when possible, or from high-quality casts, as was necessary for BAR 1002′00 ( Supplementary Table S3 ). Other partial proximal femora of Miocene apes, such as those of Morotopithecus [20] (cast of MUZM 80, kindly provided by Laura MacLatchy) and Nacholapithecus [22] , were examined but excluded from this analysis as they do not share enough common landmarks with BAR 1002′00. Geometric morphometric analyses Coordinate x, y, z data were collected from 13 points on the proximal femur using a Microscribe 3DX digitizer ( Supplementary Fig. S2 and Supplementary Table S1 ). These landmarks were selected to fully capture regions of the proximal femur that have been shown to be functionally important and that are available in BAR1002′00. Shape data were obtained from raw coordinates through a full (generalised) Procrustes fit analysis—which rotates, translates and size-scales the landmark configurations to unit of CS—and posterior orthogonal projection onto the tangent space [56] . Major patterns of shape variation among extant anthropoids in the proximal femur were inspected through PCA on the Procrustes-aligned coordinates of the extant genera mean configurations (that is, the eigenanalysis is carried out on the group means) employing the covariance matrix. To take into account the intraspecific variation of the extant samples, PC scores for all the original individuals were computed a posteriori using vector products. The method, also called ‘between-group PCA’, is extensively explained elsewhere [57] . Shape changes along the PC axes were computed by warping (using thin-plate spline) a single 3D model of the BAR 1002′00 femur along the different PCs using the Landmark Editor [58] . To facilitate visualizing the shape changes in the landmark configuration, warped surfaces in opposite extremes of every axis were superimposed for inspection using the global registration function in Geomagic (ver. 12), which applies automatic adjustments to the spatial position of two three-dimensional surfaces on the basis of all their vertices. Covariation of proximal femoral shape and size (that is, allometry) was inspected by means of multivariate regression of all the Procrustes coordinates on log-transformed CS of our 3D coordinate configuration using both extant genera/fossil species means (TIPS) and phylogenetic independent contrasts (PICS) [59] . A permutation test (10,000 rounds) against the null hypothesis of independence between the dependent (femoral shape) and independent (log CS) variables was performed in each case. To test the presence of phylogenetic signal in our morphometric data as well as to assess the phylogenetic patterning in the shape space, we used a permutation approach developed by Laurin [60] and posteriorly extended for multivariate analysis of coordinate data by Klingenberg and Gidaszewski [34] , which simulates the null hypothesis of complete absence of phylogenetic structure among proximal femoral shape on terminal taxa. The species mean shape configurations were randomly distributed as the tips of the phylogeny in 100,000 permutation rounds. For each permutation, tree length (that is, the sum of the squared Procrustes distances between ancestral and descendant shapes for all branches) was computed. If the resulting tree length computed for each permutation was greater than the one obtained with the original data, the null hypothesis of absence of phylogenetic structure in our data was rejected. The phenotypic history of the proximal femoral shape variation in extant and fossil hominoids was inspected by reconstructing hypothetical ancestral states using squared-change parsimony [30] with a method developed for geometric data in which shape is treated as a single multidimensional character and weighting by branch lengths [34] . Subsequently, the estimated ancestral node configurations were plotted on the original shape space, and the branches of the tree were connected to obtain a phylomorphospace allowing exploration of changes in hominoid proximal femur evolution. Phylogenetic trees The phylogeny used to test the presence of phylogenetic signal among extant anthropoid taxa was based on the consensus tree downloaded from 10 kTree Website (ver.3; http://10ktrees.fas.harvard.edu/ ) [61] and modified with Mesquite [62] to condense the tips at the generic level. A phylogenetic analysis including the extant and fossil hominoid taxa analysed in this study is not available. Moreover, controversy exists around the phylogenetic position of the Miocene taxa. To take into account the different phylogenetic interpretation of these fossils, we used a supertree approach, using matrix representation with parsimony (MRP) [63] , to obtain an estimation of the relationships between these fossils and the extant taxa, and thus be able to estimate plausible ancestral morphologies based on our coordinate data. Therefore, phylogenetic analyses or interpretations that include different combinations of the fossils and extant taxa incorporated here are those of Rossie and MacLatchy's (their Fig. 9a) [64] , Begun et al. [65] (their Fig. 9), Pérez de los Ríos et al. [66] (their Fig. 6 ) and Strait et al. [67] (their Fig. 10). Orrorin was situated as the first branch after the split of hominins and Pan , following the common inference of its early hominin status (for example, ref. 10 ). Trees of these previous studies were converted into MRP matrices using Mesquite [62] , and the supertree was calculated using the heuristic search option in PAUP across 10,000 rounds (random addition sequence, TBR branch swapping). The timescale for extant hominoids was extracted from a recent study based on a concatenation of 69 nuclear gene segments and 10 mitochondrial gene sequences [68] , whereas, for fossils species, estimated age for the oldest attributed fossil in the analysis ( Supplementary Table S3 ) was used. As a criterion of standardization, ghost lineages were minimized to one million years when possible (for example, not possible in the case of polytomies, resolved by introducing branches of length 0, and for Orrorin, with and estimated age very close to the Pan-Homo split). For Miocene apes, a single fossil specimen represents each species. For hominins, Australopithecus afarensis includes AL 288-1 (‘Lucy’) and AL 333-3, Paranthropus robustus includes SK 82 and SK 97, early Homo includes only KNM-ER 1481 because KNM-ER 1472 has a pathologic anterior portion of the greater trochanter and H. ergaster includes KNM-WT 15000. KNM-ER 1503 was not included in the tree due to its taxonomic uncertainty. Functional analyses The biomechanical neck length (right angle distance between the most lateral point of the greater trochanter to its most cephalad point of the femoral head) [32] was approximated by the distance between the most lateral aspect of the greater trochanter to the medial aspect of the femoral head subtracting half of head [6] . The first measure was derived from our coordinates 10 and 1, respectively; head diameter was calculated as the distance between coordinates 2 and 4. Head size was approximated by the CS of coordinates 1–6 relative to neck height, the latter computed as the distance between coordinates 7 and 8 (see Supplementary Fig. S2 for details on our coordinates). Boxplots were provided for head size relative to neck height and biomechanical neck length relative to proximal femur size (approximated by the CS) in our comparative sample. Analyses of variance (ANOVA) were provided for each analysis, and post hoc multiple comparisons were performed using the Bonferroni method. All the statistical analyses were carried out using MorphoJ [69] (ver. 1.05) and SPSS (ver. 17). How to cite this article: Almécija, S. et al. The femur of Orrorin tugenensis exhibits morphometric affinities with both Miocene apes and later hominins. Nat. Commun. 4:2888 doi: 10.1038/ncomms3888 (2013).